Identification of recurrentUSP48andBRAFmutations in Cushing’s disease Cushing’s disease results from corticotroph adenomas of the pituitary that hypersecrete adrenocorticotropin (ACTH), leading to excess glucocorticoid and hypercortisolism. Mutations of the deubiquitinase gene USP8 occur in 35–62% of corticotroph adenomas. However, the major driver mutations in USP8 wild-type tumors remain elusive. Here, we report recurrent mutations in the deubiquitinase gene USP48 (predominantly encoding p.M415I or p.M415V; 21/91 subjects) and BRAF (encoding p.V600E; 15/91 subjects) in corticotroph adenomas with wild-type USP8 . Similar to USP8 mutants, both USP48 and BRAF mutants enhance the promoter activity and transcription of the gene encoding proopiomelanocortin (POMC), which is the precursor of ACTH, providing a potential mechanism for ACTH overproduction in corticotroph adenomas. Moreover, primary corticotroph tumor cells harboring BRAF V600E are sensitive to the BRAF inhibitor vemurafenib. Our study thus contributes to the understanding of the molecular mechanism of the pathogenesis of corticotroph adenoma and informs therapeutic targets for this disease. Cushing’s disease is caused by the hypersecretion of adrenocorticotropin (ACTH) from pituitary corticotroph adenomas [1] . Chronic elevation of ACTH stimulates the adrenal glands to secrete excessive glucocorticoids, which subsequently induces hypercortisolism [2] , [3] . Cushing’s disease is a severe disease, and when left untreated, patients may develop cardiovascular disease, catabolic symptoms, hypersensitivity to infections, and mood disorders. Cushing’s disease has a prevalence of 39 cases per million of population [4] , [5] . The diagnosis of hypercortisolism and preoperative localization of the adenoma in this disease are complicated and sometimes difficult. Currently, the first-line treatment for this disease is pituitary adenomectomy. Only 65–90% of patients achieve complete or partial remission after initial transsphenoidal surgery [6] . A substantial proportion of patients tend to recur after a period of remission. It is ineffective in the treatment of patients with residual excess cortisol due to recurrent tumors or incomplete removal of tumor tissues, and no targeted therapy is currently available. So far, there has been limited genome-level study of mutations in corticotroph adenomas, hampering the development of diagnostic and therapeutic approaches for Cushing’s disease. Recently, the deubiquitinase gene USP8 was found to be mutated in 35–62% of corticotroph adenomas, resulting in sustained activation of the epidermal growth receptor (EGFR), the mitogen-activated protein kinase (MAPK) pathway, and subsequent overproduction of ACTH [7] , [8] . Inhibition of the USP8 pathway has been suggested as a targeted therapeutic strategy for the treatment of patients with USP8 -mutated adenomas [9] , [10] . Exome-sequencing studies also revealed some potential genetic lesions closely related to the pathogenic mechanism in USP8 wild-type corticotroph adenomas, including loss-of-function mutations of the glucocorticoid receptor gene NR3C1 [7] , [8] , [11] , a critical negative regulator of ACTH production. However, these studies included only a small number of corticotroph adenomas with wild-type USP8 . The genetic basis for the development of USP8 wild-type corticotroph adenomas has not yet been fully identified. In this report, we reveal recurrent mutations in the deubiquitinase gene USP48 and BRAF in corticotroph adenomas with wild-type USP8 . Similar to USP8 mutants, both USP48 and BRAF mutants enhance the promoter activity and transcription of the gene encoding proopiomelanocortin (POMC), which is the precursor of ACTH. Our study thus contributes to the understanding of the molecular mechanism of the pathogenesis of corticotroph adenoma and informs therapeutic targets for this disease. Somatic USP48 and BRAF mutations in Cushing’s disease To gain further insight into the molecular mechanisms of the pathogenesis of USP8 wild-type corticotroph adenomas, we conducted exome-sequencing of 22 paired tumor tissues and peripheral blood samples. 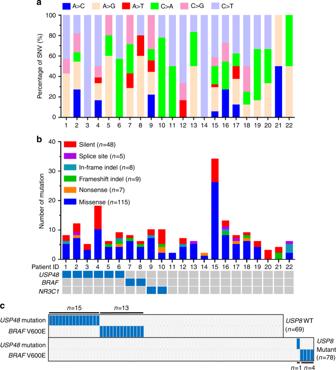Fig. 1 Whole-exome sequencing and targeted sequencing in corticotroph adenomas.aPercentage of non-silent somatic SNVs identified by whole-exome sequencing in 22 subjects with corticotroph adenomas carrying wild-typeUSP8.bThe number and type of somatic mutations identified by whole-exome sequencing (top). The mutational status of the indicated genes in each patient is shown at the bottom.cMutation frequency of the indicated genes in corticotroph adenomas with wild-type or mutatedUSP8by targeted sequencing. Each column represents a single case.n: number of subjects. Patients with the indicated mutations are marked in blue (b, c) The mean sequencing depth was 131× for the tumor samples and 95× for matched blood samples, with >10× coverage for 93.9% of tumor samples and 94.4% of blood samples (Supplementary Figure 1 ). We observed a preference for C > T/G > A alterations analogous to the somatic single-nucleotide variation (SNV) spectrum (Fig. 1a ). Next, we used deconstructSigs [12] to identify the mutational signatures of our samples. Mutation Signature 1A is associated with the SNV spectrum found in these tumors, characterized by the prominence of C > T substitutions at the NpCpG trinucleotides [13] . CpG dinucleotide is the main mutational hot-spot in most human cancers. Some C > T mutations occurred at the CpG sites. We identified a total of 144 candidate non-silent somatic mutations among the 22 cases, including 115 missense, seven nonsense, five splice-site, and 17 insertion or deletion (indel) mutations, resulting in an average of 7 (ranging from 2 to 34) somatic mutations in the exon regions (Fig. 1b and Supplementary Data 1 ). Fig. 1 Whole-exome sequencing and targeted sequencing in corticotroph adenomas. a Percentage of non-silent somatic SNVs identified by whole-exome sequencing in 22 subjects with corticotroph adenomas carrying wild-type USP8 . b The number and type of somatic mutations identified by whole-exome sequencing (top). The mutational status of the indicated genes in each patient is shown at the bottom. c Mutation frequency of the indicated genes in corticotroph adenomas with wild-type or mutated USP8 by targeted sequencing. Each column represents a single case. n : number of subjects. Patients with the indicated mutations are marked in blue ( b, c ) Full size image From this analysis, we identified four recurrently-mutated genes, including BRAF , the deubiquitinase gene USP48, NR3C1 , and host cell factor C1 ( HCFC1 ) (Fig. 1b and Supplementary Table 1 ). NR3C1 mutation has previously been discovered in corticotroph adenomas [7] , [14] . BRAF and USP48 mutations have never been reported to be related to this disease yet. 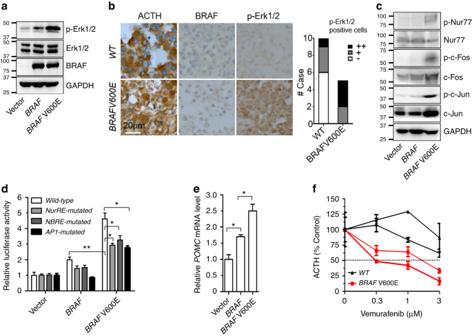Fig. 2 BRAFV600E promotesPOMCpromoter activity and ACTH production.aImmunoblotting analysis of p-Erk1/2 and total Erk1/2 in AtT-20 stably infected with wild-typeBRAForBRAFV600E.bImmunohistochemical study of p-Erk1/2 in tumor samples according to the mutational status ofBRAF. Scale bars, 20 μm.P-value was calculated using two-tailed Fisher’s exact test (P=0.036).cImmunoblotting analysis of indicated proteins in AtT-20 cells as described ina.dActivities of wild-type or various mutatedPOMCpromoters in cells transfected with wild-typeBRAForBRAFV600E together with a control vector expressing renilla luciferase.Y-axis: ratio of luciferase activity/renilla activity, presented as the means of three experiments and expressed relative to empty control vector. Error bars represent SEM of three measurements.eRelative mRNA levels ofPOMCin AtT-20 cells stably infected with indicated constructs. Data are expressed relative to the empty control vector after normalization to Hprt. Error bars represent standard SEM of three measurements. *P< 0.05, **P< 0.01, two-tailed Student’st-test (d, e).fThe inhibitory effect of vemurafenib on ACTH production in primary cultured human corticotroph adenomas (two wild-type and twoBRAFV600E). ACTH levels in culture media were measured by radioimmunoassay and presented as % of the control media. Error bars indicate SEM of three replicates. The dashed line represents IC50 We validated these recurrent mutations by Sanger sequencing (Supplementary Figure 2 ). 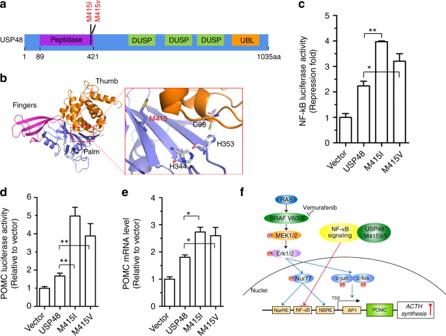Fig. 3 USP48mutants potentiatePOMCpromoter activity and ACTH production.aSchematic diagram ofUSP48domains and location of the M415 residue. DUSP, domain presents in ubiquitin-specific proteases; UBL, ubiquitin-like domain.bThe modeling structure of peptidase domain of USP48. The crystal structure of USP7 (PDB ID: 1NBF) ubiquitin aldehyde (ubal)-binding form was used as the template to build the 3D structure of peptidase of USP48. The M415 residue is located in the catalytic palm, and three catalytic triads (C98, H344, and H353) are shown.c, dThe NF-κB reporter (c) orPOMCpromoter (d) activities in cells transfected with indicated expression vectors together with control vectors expressing renilla and luciferase. Data are ratios of luciferase activity/renilla activity and presented as the mean of three experiments.eRelativePOMCmRNA levels in AtT-20 cells stably infected with indicated expression constructs. Data are expressed relative to empty control vectors after normalization to Hprt. Error bars represent SEM of three measurements. *P< 0.05, **P< 0.01, two-tailed Student’st-test (c–e).fSchematic representation showing the mechanisms by whichBRAFV600E andUSP48mutants promotePOMCtranscription in corticotroph adenomas Six of the 22 tumors had mutations in USP48 (four encoding p.M415I and two encoding p.M415V), and two of the 22 cases had BRAF mutations encoding p.V600E (Supplementary Figure 3 ). We next examined the prevalence of USP48 and BRAF mutations in additional corticotroph adenomas with wild-type USP8 by targeted sequencing. Combining the data from whole-exome and targeted sequencing, which included a total of 91 samples, we found that 16.5% of the cases (15/91) had BRAF V600E mutations and 23.1% of the cases (21/91) harbored USP48 mutations. Among the 21 USP48 -mutated cases, 11 cases had the M415I mutation and four cases harbored the M415V mutation (Supplementary Table 2 ). In addition, we sequenced USP48 and BRAF in 78 corticotroph adenomas with mutated USP8 . In contrast, only four cases had BRAF mutations (5.1%) and one case had a USP48 mutation (1.2%) (Fig. 1c ). Within a total of 169 cases, USP8 mutations are exclusive from mutations in either USP48 or BRAF in all the 169 cases ( P = 1.208 × 10 −5 and P = 0.027 receptively, two-tailed Fisher’s exact test). However, USP48 and BRAF mutations are not mutually exclusive (Fig. 1c ) ( P > 0.05, two-tailed Fisher’s exact test). We next sought to investigate whether similar mutation patterns were also present in other types of pituitary adenomas. Strikingly, none of the samples, including 20 growth hormone-secreting, 20 prolactin-secreting, and 20 non-functioning adenomas, carried either USP48 or BRAF mutations (Supplementary Figure 3 ). Therefore, similar to USP8 , BRAF and USP48 mutations appear to be unique genetic signatures of corticotroph adenomas. Functional characterization of BRAF V600E mutants It has been well established that BRAF V600E results in constitutive activation of the BRAF kinase activity and its downstream MAPK pathway in many types of human cancers [15] , [16] . BRAF is indispensible for c-AMP dependent MAPK activation. However, it has not been detected in AtT-20 cells. When we ectopically expressed BRAF V600E in a murine cell line of corticotroph adenoma (AtT-20), we observed elevated phosphorylation of Erk1/2, an indicator of MAPK activation, compared to cells with wild-type BRAF expression (Fig. 2a ). In addition, immunohistochemical analysis demonstrated that corticotroph adenomas carrying the BRAF V600E mutation had higher MAPK activity, as indicated by increased phosphorylation of Erk1/2 in these tumors compared to wild-type cases (Fig. 2b ). Fig. 2 BRAF V600E promotes POMC promoter activity and ACTH production. a Immunoblotting analysis of p-Erk1/2 and total Erk1/2 in AtT-20 stably infected with wild-type BRAF or BRAF V600E. b Immunohistochemical study of p-Erk1/2 in tumor samples according to the mutational status of BRAF . Scale bars, 20 μm. P -value was calculated using two-tailed Fisher’s exact test ( P = 0.036). c Immunoblotting analysis of indicated proteins in AtT-20 cells as described in a . d Activities of wild-type or various mutated POMC promoters in cells transfected with wild-type BRAF or BRAF V600E together with a control vector expressing renilla luciferase. Y -axis: ratio of luciferase activity/renilla activity, presented as the means of three experiments and expressed relative to empty control vector. Error bars represent SEM of three measurements. e Relative mRNA levels of POMC in AtT-20 cells stably infected with indicated constructs. Data are expressed relative to the empty control vector after normalization to Hprt. Error bars represent standard SEM of three measurements. * P < 0.05, ** P < 0.01, two-tailed Student’s t -test ( d, e ). f The inhibitory effect of vemurafenib on ACTH production in primary cultured human corticotroph adenomas (two wild-type and two BRAF V600E). ACTH levels in culture media were measured by radioimmunoassay and presented as % of the control media. Error bars indicate SEM of three replicates. The dashed line represents IC 50 Full size image We next explored critical Erk1/2 targets that could mediate the effect of BRAF V600E. Nur77 is a key transcription activator of POMC through direct binding to the Nur77-binding response element (NBRE) and Nur77 response element (NurRE) in the POMC promoter region [17] , [18] , [19] (Supplementary Figure 4 ). In addition, POMC transcription can also be induced by the c-Jun/c-Fos heterodimer, which acts by binding to the canonical AP1 binding site in the first exon of POMC [20] , [21] (Supplementary Figure 4 ). Activation of the MAPK pathway could stimulate the phosphorylation and transcriptional activation of the transcriptional regulators Nur77 [22] , c-Jun, and c-Fos [23] . As expected, we revealed that BRAF V600E expression induced phosphorylation of Nur77, c-jun, and c-fos in the AtT-20 cells (Fig. 2c ). Immunohistochemical analysis further proved that BRAF -mutated, but not wild-type corticotroph adenomas were positive for phosphorylation of Nur77, c-jun, and c-fos (Supplementary Figure 5 ). Next, using luciferase reporter assays, we showed that the introduction of wild-type BRAF , as compared to the vector control, resulted in stimulatory activity of the POMC promoter, and BRAF V600E obviously potentiated this effect (Fig. 2d ). Furthermore, the stimulatory effect of BRAF V600E on activities of the NurRE-, NBRE-, or AP1-mutated POMC promoters was considerably impaired (Fig. 2d ). Finally, ectopic expression of BRAF V600E in AtT-20 cells resulted in a substantially increased level of POMC mRNA compared to cells with wild-type BRAF (Fig. 2e ). Compared to tumor cells with wild-type BRAF , tumor cells with BRAF V600E displayed a greater reduction of ACTH secretion in response to vemurafenib, with an approximate half-maximal inhibitory concentration (IC50) of 0.3 μM, within the range of IC50 values reported for vemurafenib-sensitive tumor cells (Fig. 2f ). Moreover, vemurafenib treatment did not cause more cell death in tumors with BRAF V600E than wild-type (Supplementary Figure 6 ). These results supported the potential efficacy of vemurafenib in the treatment of corticotroph adenomas with the BRAF V600E mutation. Taken together, these results indicate that BRAF V600E contribute to the pathogenesis of ACTH-secreting pituitary adenomas through increased phosphorylation of POMC transcription regulators including Nur77, c-jun, and c-fos. Functional characterization of USP48 mutants Missense mutations of USP48 , including M415I/V substitutions, were also identified as most frequent mutations in USP8 wild-type corticotroph adenomas. Immunohistochemical analysis of USP48 protein in a series of corticotroph adenomas revealed that there was no degradation or enhanced expression of USP48 in USP48 -mutated tumors compared to tumors with wild-type USP48 (Supplementary Figure 7 ). The M415 residue was mapped to the peptidase domain of USP48 protein (Fig. 3a ) and at well-conserved amino acid positions across distinct species (Supplementary Figure 8 ). Molecular modeling further revealed that the M415 residue was spatially located in the catalytic palm of USP8 protein and inferred to be involved in regulating its catalytic activity (Fig. 3b ). We next searched for the molecular mechanisms underlying USP48 mutation-mediated POMC transcription. We first examined whether USP48 mutants activate similar signaling pathways as BRAF V600E. Western blot analysis showed that the M415I/V mutants were not able to promote phosphorylation of Erk1/2, Nur77, c-jun, and c-fos (Supplementary Figure 9 ). Immunohistochemistry also proved that USP48 -mutated corticotroph adenomas were negative or weakly positive for the phosphorylation of these molecules (Supplementary Figure 5 ). Collectively, these results demonstrate that the molecular mechanisms underlying USP48 mutation-mediated POMC transcription do not involve Erk1/2 or its downstream signaling cascade. Fig. 3 USP48 mutants potentiate POMC promoter activity and ACTH production. a Schematic diagram of USP48 domains and location of the M415 residue. DUSP, domain presents in ubiquitin-specific proteases; UBL, ubiquitin-like domain. b The modeling structure of peptidase domain of USP48. The crystal structure of USP7 (PDB ID: 1NBF) ubiquitin aldehyde (ubal)-binding form was used as the template to build the 3D structure of peptidase of USP48. The M415 residue is located in the catalytic palm, and three catalytic triads (C98, H344, and H353) are shown. c, d The NF-κB reporter ( c ) or POMC promoter ( d ) activities in cells transfected with indicated expression vectors together with control vectors expressing renilla and luciferase. Data are ratios of luciferase activity/renilla activity and presented as the mean of three experiments. e Relative POMC mRNA levels in AtT-20 cells stably infected with indicated expression constructs. Data are expressed relative to empty control vectors after normalization to Hprt. Error bars represent SEM of three measurements. * P < 0.05, ** P < 0.01, two-tailed Student’s t -test ( c–e ). f Schematic representation showing the mechanisms by which BRAF V600E and USP48 mutants promote POMC transcription in corticotroph adenomas Full size image USP48 has been implicated in the activation of NF-κB [24] , [25] , which directly binds to the promoter of POMC and participates in regulating its transcription in AtT-20 cells [26] . We examined whether USP48 mutation affects its interaction with RelA, a subunit of NF-κB. As shown in Supplementary Figure 10 , the M415I/V mutants retained the ability to interact with RelA. Then we conducted luciferase reporter assays to evaluate the effect of M415I/V alteration on the activity of USP48 protein. USP48 M415I/V mutants had a greater inhibitory effect on the activity of NF-κB reporter than wild-type USP48 , indicating gain-of-function of the M415I/V mutation (Fig. 3c ). We also demonstrated that overexpression of wild-type USP48 had a minor stimulatory effect on the POMC promoter activity compared to the control vector; however, this effect was markedly potentiated by either M415I or M415V mutants (Fig. 3d ). Finally, the mRNA abundance of POMC was higher in AtT-20 cells stably transfected with USP48 M415I/V than in cells with wild-type USP48 (Fig. 3e ). Clinical phenotypes and mutational status We previously reported that USP8 -mutated corticotroph adenomas are small in size and have higher ACTH production. Thus, we explored whether patients with BRAF V600E or USP48 -mutated tumor display distinct clinical features. Patients with BRAF V600E had significantly higher levels of midnight plasma ACTH ( P = 0.023, Mann–Whitney U -test) and midnight serum cortisol ( P = 0.007, Mann–Whitney U -test) (Table 1 ), but similar tumor sizes, when compared with patients carrying wild-type BRAF / USP48 . Therefore, BRAF V600E appears to promote ACTH production. Other clinical features examined are undistinguished between patients with wild-type BRAF and BRAF V600E. Patients with USP48 -mutated tumors have quite similar clinical features as those with wild-type BRAF / USP48 . Table 1 Clinical and phenotypic features of patients with Cushing’s disease Full size table Recently, two exome sequencing studies suggested the presence of mutations in the USP8 genes of 35–62% of people with corticotroph adenomas [7] , [8] . However, the potential genetic risk of USP8 wild-type corticotroph adenomas remains unknown. Here, we performed further exome sequencing and identified recurrently-mutated genes including BRAF and USP48 in USP8 wild-type corticotroph adenomas. Corticotroph adenomas showed a preference for C > T mutation, and some of these alterations occurred at the CpG sites. The C of CpG is a preferential site of methylation, and the methyl-C is prone to spontaneous deamination to T [27] . This is the most likely reason for CpG dinucleotide to be the main mutation hot-spot in most human cancers. Therefore, it is not surprising that corticotroph adenomas have this mutation spectrum. These results provide a comprehensive genetic landscape for this tumor. We found that mutations in USP48 and BRAF were also key genetic lesions of Cushing’s disease. Six of the 22 tumors had mutations in USP48 (p.M415I or p.M415V) and two of the 22 cases had BRAF mutations (p.V600E) by exome sequencing. We screened the prevalence of USP48 and BRAF mutations in additional 69 corticotroph adenomas with wild-type USP8 . We found that 18.8% of these cases (13/69) had BRAF V600E mutations and 21.7% of these cases (15/69) harbored USP48 mutations. However, neither BRAF V600E nor USP48 M415I/M415V was detected in other types of pituitary adenomas. Therefore, similar to USP8 , BRAF and USP48 mutations appear to be unique genetic signatures of corticotroph adenomas. We assumed that mutations in BRAF and USP48 should be involved in the pathogenesis of corticotroph adenomas. BRAF V600E represents a mutational hotspot in melanomas [15] , craniopharyngioma [28] , and multiple types of cancers [15] , [28] , [29] , [30] , [31] , [32] , and its oncogenic activity has been extensively characterized [15] , [28] , [29] , [30] , [31] , [32] . In our study, an elevated kinase activity of BRAF V600E compared to wild-type BRAF was observed in corticotroph adenomas just like in other types of tumors, leading to activation of MAPK pathway and transactivation of POMC, which is the precursor of ACTH. Deregulated MAPK signaling is frequently observed in corticotroph adenomas, promoting ACTH production [33] , [34] . Previous studies have demonstrated that the USP8 mutation causes corticotroph adenomas mainly through activating the EGFR–MAPK signal cascades [7] , [8] . Orphan nuclear receptor Nur77 acts as a mediator of corticotrophin-releasing hormone (CRH)-induced POMC transcription and plays an important role in the hypothalamic–pituitary–adrenal axis. In addition, POMC transcription can also be induced by the c-Jun/c-Fos heterodimer, which acts by binding to the canonical AP1-binding site in the first exon of POMC [20] , [21] (Supplementary Figure 4 ). Activation of the MAPK pathway could stimulate phosphorylation and transcriptional activation of the transcriptional regulators Nur77 [22] , c-Jun, and c-Fos [23] . Collectively, our results demonstrated that Nur77 and the c-Jun/c-Fos heterodimer mainly mediate the stimulatory effect of BRAF V600E on POMC transcription. We next sought to evaluate the effect of the BRAF inhibitor vemurafenib on ACTH secretion in primary human corticotroph adenomas. The results supported the potential efficacy of vemurafenib in the treatment of corticotroph adenomas with the BRAF V600E mutation. Of note, although both corticotroph adenomas and craniopharyngioma are pituitary tumors, and share some common clinical features, it is generally believed that they have different cellular origins. Considering the fact that BRAF V600E has been detected in many types of brain tumors, the observation that corticotroph adenomas and craniopharyngioma [28] have BRAF V600E appears not to be the evidence to support any connection between these tumor types. Missense mutations of USP48 , including M415I/V substitutions, were found at a very low frequency in several types of human cancers in the available cancer data sets, and its biological significance in tumors has not been fully described [35] . A luciferase report assay showed that USP48 M415I/V promoted the POMC promoter activity. Moreover, the higher mRNA abundance of POMC in AtT-20 cells stably transfected with USP48 M415I/V, further supports the notion that the M415I/V substitution causes corticotroph adenomas by up-regulating POMC transcription. Different from BRAF V600E, USP48 mutation-mediated transcriptional activation of POMC appears not be linked to the activation of Erk1/2 or its downstream signaling cascade. In contrast, we provide the evidence to demonstrate that the NF-κB pathway is involved in USP48 -mediated transcriptional activation of POMC . Several cytokines and hormones, including CRH, were reported to induce transcriptional activation of the pituitary POMC gene by directly suppressing NF-κB activity in AtT-20 cells [26] . AtT-20 cells displayed constitutive NF-κB activation, and inhibition of NF-κB activity increased transcription of the POMC gene. Moreover, USP48 has been implicated in the activation of NF-κB [24] , [25] . Accordingly, USP48-mediated inhibition of NF-κB activity could promote the transcription of POMC gene. However, these USP48 mutants also promoted the activity of NF-κB binding site-mutated POMC promoters (Supplementary Figure 11 ), suggesting the existence of alternative USP48 substrates involved in the transcriptional control of POMC . It is very likely that USP8 mutation activates the transcription of POMC via multiple pathways including the NF-κB pathway. Further studies are needed to reveal the underlying molecular mechanisms. In summary, our study identified frequent BRAF and USP48 mutations in corticotroph adenomas carrying wild-type USP8 and indicated that these mutations cause Cushing’s disease mainly by activating POMC gene transcription and increasing plasma ACTH levels (Fig. 3f ). ACTH overproduction is a hallmark of Cushing’s disease and appears to be frequently induced by mutations in genes that tightly regulate POMC gene transcription in the pathogenesis of this disease. This concept is further supported by the observation that except for USP8 , BRAF, and USP48 , there were detectable somatic mutations in genes that potentially affect MAPK signaling and POMC transcription. These mutated genes include serum response factor ( SRF ) and PPP2R5D , which were detected in individual tumor samples (Supplementary Data 1 ). Similar to the USP8 mutation, BRAF V600E and USP48 M415I/V were not detected in other types of pituitary adenomas, highlighting their specificity for corticotroph adenomas. Unlike malignant tumors, benign pituitary adenomas, including corticotroph adenomas, have a relatively low number of somatic mutations per tumor, suggesting that each mutation found in a pituitary adenoma has a higher chance to be a driver mutation and might have a profound effect on its pathogenesis. The mutational status of BRAF, USP8 , and USP48 in corticotroph adenomas may be used in the future to characterize the molecular subtypes and guide targeted molecular therapy. Our findings suggest an immediately operable drug target for corticotroph adenomas carrying BRAF V600E. Study patients Patients were recruited for this study at the Department of Neurosurgery in Huashan Hospital affiliated to Shanghai Medical College, Fudan University from 2003 to 2016. A total of 229 patients (91 with USP8 -WT ACTH-secreting adenomas, 78 with USP8 -mutated ACTH-secreting adenomas, 20 with growth hormone-secreting adenomas, 20 with prolactin-secreting adenomas, and 20 with non-functioning adenomas) were included in this study. This study was approved by the ethics committee of Huashan Hospital and informed consent was obtained from each patient. Cushing’s disease was diagnosed according to the clinical manifestations, endocrine laboratory tests and imaging [8] , and was histologically confirmed after surgical resection. Whole-exome sequencing A DNeasy Blood and Tissue DNA isolation kit (Qiagen) was used to extract genomic DNA from freshly frozen tumors and peripheral blood samples. An ultrasonicator Covaris E-220 (Covaris) was used to randomly fragment genomic DNA to 200–300 bps in size. We used Agencourt AMPure XP beads (Beckman) to purify the DNA and then ligated adaptors with sample-specific barcodes at both ends. The adapter-ligated products were purified using beads and amplified by ligation-mediated PCR. A TruSeq TM Exome Enrichment Kit and an Agilent SureSelect Human All Exon V5+UTR Kit (Agilent) was used to capture exome-enriched DNA fragments. Then, Agilent 2100 was used to estimate the magnitude of enrichment. Each library was loaded on the HiSeq 2500 platform for sequencing. Bioinformatic analysis Raw sequencing reads were filtered with trimmomatic ( http://www.usadellab.org/cms/index.php?page=trimmomatic ) and mapped to the reference hg19 human genome with Burrows-Wheeler Aligner (BWA) 0.7.7. PCR duplicates were removed with MarkDuplicates tool from Picard ( http://picard.sourceforge.net ), and then locally realigned using the Indel Realignment and recalibrated using the BaseRecalibrator tool from GATK. Somatic single-nucleotide variants (SNVs) were detected using MuTect v1.1.7 and VarScan 2, while somatic indels were identified using VarScan 2 and Genome Analysis Toolkit Somatic indel detector with default parameters. The set of mutations passed by somatic caller was dropped into post-processing filters to reduce false positive calls. Filter criteria for high-confidence were as follows: (1) a minimum depth of 5× in both tumors and their normal pairs; (2) reads depth of variant alleles in tumors should be more than 4×, and with read quality of 20; (3) to avoid artifacts and likewise enable calling more variants on sites with lower error rates, somatic variants were filtered for allele frequencies greater than 10%. Filtered somatic mutations were manually reviewed for accuracy using Integrative Genomics Viewer (IGV, Broad Institute, Cambridge, MA, USA). All high-quality somatic mutations were annotated based on the information available in catalog of somatic mutations in cancer (COSMIC; http://cancer.sanger.ac.uk/cosmic ), dbSNP138 ( http://www.ncbi.nlm.nih.gov/snp ), the 1000 Genomes Project ( http://www.1000genomes.org/ ), and EXAC ( http://exac.broadinstitute.org/ ) by Annovar. Germline variants with mutation frequencies >0.1% of the allelic fraction in these databases were removed. Mutational signatures in our study were identified by deconstructSigs [12] . Candidate gene validation SNV and indels were validated by PCR reaction and Sanger sequencing. PCR primers were designed using the online software Primer3 ( http://frodo.wi.mit.edu/primer3/ ) using GRCh37/hg19 as the reference sequence. We used a 96-well GeneAmp PCR System 9700 (Applied Biosystems) to perform the PCR reaction. A total of 10 ng of DNA from each sample was used per reaction with the 2× Taq PCR Master Mix (Vazyme Biotech). The sequencing reactions were performed with the Big Dye Terminator v.3.1 kit (Applied Biosystems). PCR products were sequenced using a 3730xl DNA Analyzer (Applied Biosystems). DNA constructs and site-directed mutagenesis Full-length wild-type cDNA of human USP48 and BRAF were cloned into the lentivirus expression vector pCDH-EF1-MCS-T2A-Puro (System Biosciences). The desired mutations in BRAF and USP48 cDNA were introduced using a QuikChange II Site-Directed Mutagenesis Kit (Agilent Technologies). The primers used in the construction of cDNA expression plasmids and mutagenesis are listed in Supplementary Table 3 . Homology modeling A Blast search was used to search for homologs of USP48. The crystal structure of USP7 (PDB ID:1NBF [36] ) ubiquitin aldehyde (ubal)-binding form was used as the template to build the 3D structure of USP48 by “Build Homology Models” module of Discovery studio 4.0 software (Accelrys, Inc., San Diego, CA). The geometrical reasonability of the modeled USP48 structure was checked with a Procheck [37] analysis. Immunohistochemistry Consecutive sections (5 μm thick) of each formalin-fixed paraffin-embedded (FFPE) tissue block were subjected to immunohistochemical staining. Briefly, the slides were deparaffinized, re-hydrated, and then immersed in distilled water with 3% hydrogen peroxidase in methanol for 20 min to suppress endogenous peroxidase activity. Sections were incubated with primary antibodies of anti-USP48 (1:200, Abcam), anti-BRAF (1:200, Abcam), anti-p-Erk1/2 (1:200, Abcam), and anti-ACTH (1:200, Abcam) at 4 °C overnight. Subsequently, an ABC staining kit (Vector Laboratories) was applied to the sections, and signals were developed with diaminobenzidine (DAB) chromogen (Vector Laboratories). The analysis of our immunohistochemical stainings is based on the evaluation method according to ref. [38] . Western blotting Cell and tumor tissues were lysed in RIPA lysis buffer (Sigma) supplemented with complete protease inhibitor cocktail (Roche). The resultant protein extracts were subjected to western blotting using a standard protocol. The following primary antibodies were used in this study: anti-actin (1:5000, Abcam); anti-USP48 (1:1000 Abcam); anti-GAPDH (1:1000, Abcam); anti-BRAF (1:1000, Abcam), anti-Erk1/2, anti-p-Erk1/2 anti-c-Fos (1:1000, Cell Signaling Technology), anti-c-Jun (1:1000, Cell Signaling Technology), anti-Nur77 (1:1000, Abcam), anti-p-c-Fos (1:1000, Cell Signaling Technology), anti-p-c-Jun (1:1000, Cell Signaling Technology), and anti-p-Nur77 (1:1000, Cell Signaling Technology). Uncropped images of the blots are provided in Supplementary Figure 12 . Dual-luciferase reporter assay For luciferase reporter assays, AtT-20 cells seeded in a 24-well plate were transiently transfected with PGL3 basic vector (Promega), together with the transfer vector. Luciferase activity was detected using the Dual-luciferase reporter assay systems (Promega) according to the manufacturer’s instructions. Chemiluminescence was measured using an EnVision Multilabel Reader (PerkinElmer, Waltham, MA, USA). Quantitative RT-PCR To determine the relative mRNA level of POMC , quantitative RT-PCR was performed as previously described [8] . RT-PCR was performed using SYBR® Premix Ex Taq™ (Tli RNaseH Plus) (TAKARA) to examine the mRNA abundance. Hypoxanthine-guanine phosphoribosyltransferase ( HPRT ) was used as an internal control to normalize the expression levels. The following primers were used: for POMC, forward 5′-GAGGCCACTGAACATCTTTGTC-3′, reverse 5′-GCAGAGGCAAACAAGATTGG-3′; for HPRT, forward 5′-ACCAGTCAACAGGGGACATAAA-3,′ reverse 5′-CTGACCAAGGAAAGCAAAGTCT-3′. Cell culture and transfection All cell lines used in this study were purchased from the American Type Culture Collection (ATCC, Manassas, VA, USA). The cell lines were routinely tested for mycoplasma contamination using the MycoAlert detection kit (Lonza). AtT-20 and HEK293 cell lines were maintained in DMEM (HyClone) supplemented with 10% fetal calf serum (FCS) at 37 °C in a humidified atmosphere with 5% CO 2 . Methods of transfection and culture of primary tumor cells derived from human ACTH-secreting pituitary adenomas were the same as previously described [8] . Transfection was performed using SuperFect Transfection Reagent (QIAGEN) according to manufacturer’s protocol. After 24 h of culture, primary human pituitary cells were incubated with the BRAF inhibitor vemurafenib (0, 0.3, 1, and 3 μM) for 48 h before analysis for ACTH secretion. Radioimmunoassay Plasma ACTH concentrations were measured by a sensitive and specific immunoradiometric assay. The sensitivity of the assay was 4.13 nmol/L for ACTH, and the inter- and intra-assay coefficients of variations were between 5–7% and 6–7.9%, respectively. The final results are expressed as picograms per milliliter. Cortisol concentrations were measured using a commercially available RIA kit (ICN Biomedicals, Inc., Costa Mesa, CA). Statistical analysis Statistical analysis was performed using SPSS version 17.0 (SPSS Inc.). Prism 6.0 (GraphPad) software was used to prepare graphs. Pearson’s χ 2 test was used for the categorical variables. The Mann–Whitney U -test was used for the continuous variables. P -values less than 0.05 were considered to be statistically significant. Data availability Sequence data have been deposited at the European Genome-phenome Archive (EGA), which is hosted by the EBI and the CRG, under accession number EGAS00001003029.